Photon diffusion near the point-of-entry in anisotropically scattering turbid media From astronomy to cell biology, the manner in which light propagates in turbid media has been of central importance for many decades. However, light propagation near the point-of-entry in turbid media has never been analytically described, until now. Here we report a straightforward and accurate method that overcomes this longstanding, unsolved problem in radiative transport. Our theory properly treats anisotropic photon scattering events and takes the specific form of the phase function into account. As a result, our method correctly predicts the spatially dependent diffuse reflectance of light near the point-of-entry for any arbitrary phase function. We demonstrate that the theory is in excellent agreement with both experimental results and Monte Carlo simulations for several commonly used phase functions. Recent advances in optical spectroscopy of human epithelium, high-resolution imaging and early cancer detection demand an accurate description of light propagation near the point where light enters the tissue [1] , [2] , [3] , [4] , [5] , [6] , [7] , [8] . However, an analytical method capable of describing the propagation of photons near their point-of-entry (POE) in turbid media has eluded researchers in diverse fields for generations [9] , [10] , [11] , [12] . Propagation of electrons in semiconductors [13] , anisotropic light diffusion in liquid crystals [14] and coherent backscattering [15] are only a few examples that can benefit from such a method. The most accurate treatment of such problems, when interference can be neglected, uses the radiative transport equation, where L ( r , s ) is the radiance of light at position r travelling in the direction of unit vector s , S ( r , s ) describes the distribution of internal sources, and μ a and μ s are the absorption and scattering coefficients of the medium, respectively. The unity normalized function p ( s , s ′) is the phase function of the medium, which describes the angular distribution for a single scattering event (here, s ′ is the incoming and s the outgoing direction of scatter) [9] . Unfortunately, no analytical solution to this equation has been discovered for practical scenarios. A frequently used numerical method is the Monte Carlo (MC) simulation. The MC simulation gives accurate results but does not provide any physical insight and often requires excessive computational time. Recent GPU-based MC methods significantly reduce computational time [16] , [17] , [18] , [19] , thus extending the utility of the MC simulations to practical applications, but inverse problems with a large number of parameters will greatly benefit from the analytical approach provided here. In the absence of suitable numerical methods, the most widely used approach is to obtain an approximate solution using the diffusion approximation (DA) to the radiative transport equation. The DA works best when scattering is isotropic or near isotropic [20] . It is not sensitive to the particular form of the phase function, reducing phase function information to a single parameter, g =∫ p ( s · s ′) ( s · s ′) d s ′, called the average cosine of the phase function or the anisotropy factor, which in turn is incorporated into the reduced scattering coefficient, . Hence, becomes the only parameter in the DA to describe scattering. Although the DA can provide analytical solutions in some cases, it does not provide accurate results for the critically important region near the POE. This limitation of the DA has been a major impediment, particularly for light scattering in biological media. Many investigators have attempted to amend the DA by solving the radiative transport equation by using more complicated phase functions [21] , [22] , [23] . One such approach, called the δ − P 1 approximation, is to solve the equation for the delta-Eddington phase function, which results in some improvements for characterizing forward scattering media [24] . Another approach is to decompose the phase function into a series of Legendre polynomials and to construct a system of radiative transport equations corresponding to each Legendre term. Because it becomes very cumbersome to solve the system of partial differential equations as the number of Legendre terms increases, the P 3 approximation uses only the 0th through 3rd terms in the Legendre series [25] . Both approximations are substantial improvements over the DA because they take the phase function into account and broaden the parameter space with which the approximation can be used [26] , [27] . However, until now, no proposed analytical method has addressed the important regime of light scattering near the POE (for example, at source–detector separations less than ) well enough to be widely used as common practice. Here we introduce a novel approach that results in the first successful attempt to analytically describe spatially dependent diffuse reflectance near the POE in turbid media with arbitrary phase function and absorption. The phase function corrected (PFC) DA takes advantage of the delta-isotropic phase function, described below, to derive a two-part expression for the diffuse reflectance. The first part is identical to the DA for a pencil beam illumination, whereas the second part approximates the changes in reflectance due to the specific form of the phase function. The resulting predictions are shown to be in excellent agreement with experiment and also with the MC simulations at all distances, including the critical area near POE. PFC photon diffusion We consider the problem of calculating the reflectance of light from a semi-infinite turbid medium with no internal sources ( S ( r , s )=0) illuminated with a narrow collimated beam ( Fig. 1 ), an important, general problem often treated using the DA. 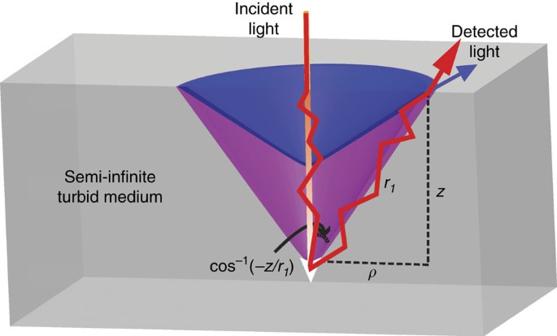Figure 1: Semi-infinite turbid medium geometry. The medium is illuminated with a narrow collimated beam. In addition to unscattered photons, low-angle-scattered photons are also shown. Any point along the beam can be a source of a single large-angle turn, which is followed by low-angle-scattered photons propagating towards the surface. The large angle turn is described by the phase function, providing PFC. Here. Figure 1: Semi-infinite turbid medium geometry. The medium is illuminated with a narrow collimated beam. In addition to unscattered photons, low-angle-scattered photons are also shown. Any point along the beam can be a source of a single large-angle turn, which is followed by low-angle-scattered photons propagating towards the surface. The large angle turn is described by the phase function, providing PFC. Here . Full size image The radiance in this problem can be divided into three main parts as follows: an on-axis part due to the narrow collimated beam; a predominately isotropic, phase function-independent part; and an anisotropic, phase function-dependent part. Similarly, any arbitrary phase function can be expressed as a sum of a delta function, an isotropic part and an anisotropic part. We achieve this by expressing an arbitrary phase function, p ( s · s ′), as the sum of the delta-isotropic phase function with the same anisotropy factor and a deviation term where p DI ( s · s ′)=[1− g +2 g · δ (1− s · s ′)]/4π is the delta-isotropic phase function [28] . This decomposition of the phase function enables us to separate the radiance into the three analogous parts described above. By substituting equation (2) into equation (1) and using the reduced scattering coefficient, we can express equation (1) as Without the second integral on the right-hand side, equation (3) would be the equation of radiative transport for the case of an isotropically scattering medium, which, as mentioned above, can be described using the DA. Thus, indeed, it is logical to present the radiance L ( r , s ) as the sum of a predominantly isotropic diffuse part, L d ( r , s ), a phase function-dependent part, L p ( r , s ), and an on-axis part due to the narrow collimated beam, L c ( r , s ). After substitution for L ( r , s ) in equation (3), we seek an expression for L c ( r , s ), which satisfies the boundary condition for a narrow collimated beam and a portion of equation (3), . Note that this portion is described by rather than μ s and specifically accounts for low-angle-scattered photons [20] (see Fig. 1 for illustration). The boundary condition corresponding to a narrow collimated beam entering a semi-infinite medium is for inward directions , where P 0 is the power of the incoming beam, ρ and z are the cylindrical coordinates and is a unit vector along the z axis. This gives [29] and the boundary conditions and for . The transport equation (3) can then be written as a system of two equations for the remaining parts of the radiance L d ( r , s ) and L p ( r , s ). It is natural then to distribute the two remaining L c ( r , s ) dependent terms so that the isotropic, phase function-independent term is combined with the equation for the predominately isotropic L d ( r , s ) and the anisotropic, phase function-dependent term μ s ∫∫[ p ( s · s ′)− p DI ( s · s ′)] L c ( r , s ′)d s ′ is combined with the equation for the anisotropic L p ( r , s ). The first equation, leads to the standard DA and the second equation, retains all of the phase function-dependent terms. Here we use μ s ∫∫[ p ( s · s ′)− p DI ( s · s ′)] L d ( r , s ′) d s ′=0 and neglect the integral term μ s ∫∫[ p ( s · s ′)−(2π) −1 g · δ (1− s · s ′)] L p ( r , s ′) d s ′. (The justification for the treatment of these two integrals appears in the Methods section.) Equation (4) exactly matches the equation of radiative transport for a turbid medium with an isotropic phase function, illuminated with a narrow collimated beam, and has been solved by a standard DA procedure. This results in the radially dependent diffuse reflectance R d ( ρ ) presented in Farrell et al ., [30] where is the effective attenuation coefficient, is the coordinate of the extrapolated boundary condition, and ρ is the exit radius measured from the POE in the surface plane of the semi-infinite medium ( Fig. 1 ). Equation (5) describes the PFC and is also integrable. The solution gives the PFC term, R p ( ρ ), for the radially dependent reflectance, obtained by projecting L p ( r , s ) on the surface of the medium and integrating over the emerging solid angle Physical nature of PFC The physical nature of the PFC in equation (7) can be qualitatively understood if we notice that z + r 1 is the distance a photon would travel through the turbid medium to the detector if it undergoes just a single scattering event, first travelling in the collimated beam to the depth z , then scattering at the angle cos −1 (− z / r 1 ) and finally travelling distance r 1 to the detector ( Fig. 1 ). Moreover, the phase function in the integral p (− z / r 1 ) represents the probability of scattering at an angle cos −1 (− z / r 1 ). However, note that the attenuation (the exponential in equation (7)) has a characteristic inverse scattering length of . The reduced scattering coefficient characterizes the attenuation of light due to diffuse scattering, that is, only diffusely scattered photons are removed from the z + r 1 path; unscattered and low-angle-scattered photons remain. If we were considering only unscattered photons, the attenuation factor would have the scattering coefficient μ s in the exponent, instead of the reduced scattering coefficient . The z + r 1 path is not the actual path of real photons, but rather the virtual path of quasi-ballistic photons, which are described by equation (7). The contribution of the term describing this behaviour can be positive or negative as it depends on the difference of the contributions of the actual phase function and the delta-isotropic phase function. Physically, the PFC term accounts for the contribution of these photons, which have undergone multiple low-angle scattering events plus a single large-angle scattering event along the z + r 1 path. That single large-angle turn is described by the phase function, thus providing the PFC. An illustration of this scattering behaviour is shown in Figure 1 . Comparison with the MC and existing approximations To check the accuracy of PFC we compared the reflectance calculated by the MC simulation, which is considered to be the gold standard, to the reflectance calculated using PFC, that is, the sum of the standard DA term, equation (6), and the PFC term, equation (7). The MC program used was validated against a well-accepted code [31] . Following the procedure described in Liu and Ramanujam [32] , we obtained the 95% confidence interval of all the MC simulations presented. The margin of error is within 1% of the mean for and within 2% for the full range. We include results for two phase functions commonly used in turbid media: the Henyey – Greenstein (H–G) phase function [33] p HG ( s · s ′)=[(1− g 2 )/4π]/[1+ g 2 −2 g ( s · s ′)] 3/2 and the 'Mie' phase function, which can be described using the Mie theory [34] . The Mie phase function was calculated for a Gaussian size distribution with a s.d. of 10% and a mean size chosen such that the resulting phase function had the desired anisotropy factor, g . The results are presented in Figures 2 and 3 . 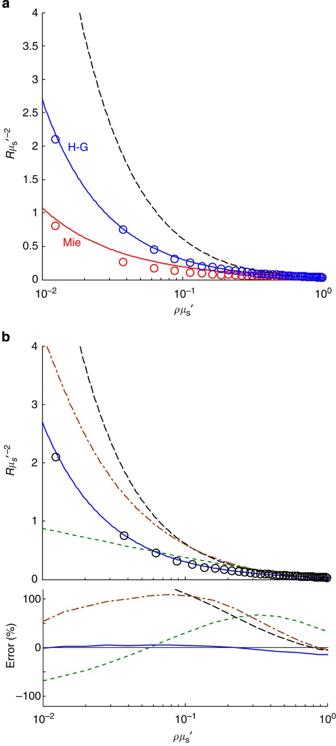Figure 2: Sensitivity to the form of the phase function and comparison with other light transport approximations. (a) Dimensionless reflectance for the H–G and Mie phase functions withg=0.95 and=0.01. Blue lines and circles—H–G phase function, red lines and circles—Mie phase function, where lines are for PFC diffusion theory and circles are for the MC simulations. Black dashed line—the standard DA. (b) Comparison of PFC diffusion theory with the standard DA, theP3andδ−P1approximations and MC simulations for the H–G phase function withg=0.95 and=0.01. The error plot shows the percentage error ((R−RMC)/RMC×100%), between each of the approximations,R, and MC simulation,RMC. Figure 2: Sensitivity to the form of the phase function and comparison with other light transport approximations. ( a ) Dimensionless reflectance for the H–G and Mie phase functions with g =0.95 and =0.01. Blue lines and circles—H–G phase function, red lines and circles—Mie phase function, where lines are for PFC diffusion theory and circles are for the MC simulations. Black dashed line—the standard DA. ( b ) Comparison of PFC diffusion theory with the standard DA, the P 3 and δ − P 1 approximations and MC simulations for the H–G phase function with g =0.95 and =0.01. The error plot shows the percentage error (( R − R MC )/ R MC ×100%), between each of the approximations, R , and MC simulation, R MC . 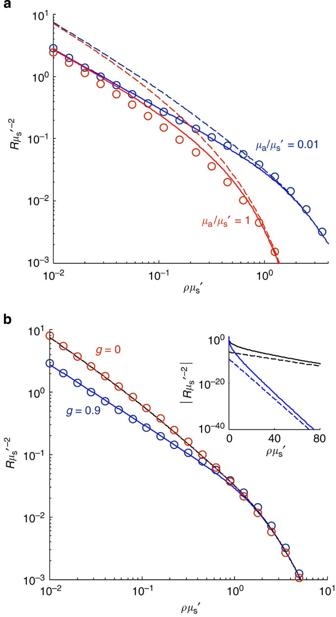Figure 3: Effects of absorption and anisotropy factorg. Dimensionless reflectance for the PFC diffusion theory compared with the MC simulations and the standard diffusion theory (DA) for the case of the H–G phase function with different absorptions; (a) blue lines and circles—g=0.9 and relatively weak absorption (), red lines and circles—g=0.9 and relatively high absorption (). Dashed lines—standard DA, solid lines—PFC diffusion theory, circles—MC simulations. Although the standard diffusion theory gives significant errors forthe PFC DA does not suffer from this problem and agrees with the MC simulations for all distances; (b) effect of different anisotropy factorsg. Red representsg=0 and blue representsg=0.9. The PFC diffusion theory (solid lines) agrees with the MC simulations (circles) for all distances, whereas the standard diffusion theory (black dashed line) does not have any dependence on the anisotropy factorg. (Note that the standard diffusion theory and the PFC diffusion theory curves exactly overlap forg=0.) Inset: the separate contributions of the diffuse reflectance (black line) and PFC reflectance (blue line) and their asymptotic behaviour (dashed lines.) Full size image Figure 3: Effects of absorption and anisotropy factor g . Dimensionless reflectance for the PFC diffusion theory compared with the MC simulations and the standard diffusion theory (DA) for the case of the H–G phase function with different absorptions; ( a ) blue lines and circles— g =0.9 and relatively weak absorption ( ), red lines and circles— g =0.9 and relatively high absorption ( ). Dashed lines—standard DA, solid lines—PFC diffusion theory, circles—MC simulations. Although the standard diffusion theory gives significant errors for the PFC DA does not suffer from this problem and agrees with the MC simulations for all distances; ( b ) effect of different anisotropy factors g . Red represents g =0 and blue represents g =0.9. The PFC diffusion theory (solid lines) agrees with the MC simulations (circles) for all distances, whereas the standard diffusion theory (black dashed line) does not have any dependence on the anisotropy factor g . (Note that the standard diffusion theory and the PFC diffusion theory curves exactly overlap for g =0.) Inset: the separate contributions of the diffuse reflectance (black line) and PFC reflectance (blue line) and their asymptotic behaviour (dashed lines.) Full size image Figure 2a shows the sensitivity of PFC to the particular choice of phase function. Although the DA strongly disagrees with the results of the MC simulations, especially in the vicinity of the source ( ), PFC shows excellent agreement for both the H–G and Mie phase functions. As an example, a comparison is presented for g =0.95, although for other values of the anisotropy factor g the agreement is equally good. Importantly, both the H–G and Mie phase functions used in these simulations have identical anisotropy factors, yet, show marked differences at small source–detector separations. As demonstrated in Figure 2a , these phase function-dependent changes in reflectance are well characterized by PFC. Comparison between PFC and recent attempts to improve the DA is shown in Figure 2b , together with a plot of the percentage error between the approximations and MC simulation. The PFC diffusion theory shows significantly improved agreement with the MC simulations over both the δ − P 1 and P 3 approximations. For the case of the Mie phase function, PFC shows similar results, although the comparison of δ − P 1 and P 3 approximations with the MC simulations demonstrate improvement compared with Henyey–Greenstein phase function close to the POE ( Supplementary Fig. S1 ). Figure 3 presents several scenarios where PFC corrects the major deficiencies of the DA. Scenarios of low and high absorption are shown in Figure 3a . The DA gives significant errors for , that is, small distances from the source; however, PFC does not suffer from this problem and agrees with the MC simulations for all distances. For large source–detector separations and high absorptions, the amount of light emerging from the scattering medium is usually so small that detection is impractical. Figure 3b shows the effects of varying the anisotropy factor g . PFC agrees with the MC simulations for both g =0 and g =0.9, whereas the DA is only accurate for anisotropy factor g =0, that is, totally isotropic scattering. Percentage errors between theory and the MC for Figure 3 are shown in Supplementary Figure S2 . The inset in Figure 3b depicts the separate contributions of R p ( ρ ) and R d ( ρ ) and their asymptotic rates of decay for the g =0.9 case. The contribution of the correction to the reflectance at becomes negligible, resulting in an accuracy that is determined by the particular diffusion theory model being used. Note that although we have chosen a well-accepted diffusion theory model to describe isotropic scattering, there may be other solutions to this component of the reflectance. The correction is intended to work best near the POE where the specific form of the phase function has a role, although the DA is known to work well for large radii where the specific form of the phase function does not matter. The intermediate regime is described less accurately due to the neglected integral term. The average deviation in this range of is less than 10%, which is significantly better than the other methods ( Fig. 2b ). Comparison with the MC simulation within the medium Though the primary intention of this work is to present a solution to the problem of diffuse reflectance near the POE, we note that the correction also works within the medium. The approach presented above uses the standard DA to provide the isotropic solution, which is then corrected with the PFC. However, the standard DA is not particularly accurate in predicting the distribution of light near the POE within the medium, even for g =0. Thus, to check the accuracy of the correction within the medium, we used the MC simulation for both isotropic and anisotropic cases using the H–G phase function and calculated the phase function-related change in the fluence rate at several depths within the medium. The PFC fluence rate is obtained by integrating L p ( r , s ) over the entire solid angle where . Comparison with the MC simulations shows good agreement within the medium including the vicinity of the POE ( Fig. 4 ) at depths of . Accurate treatment of larger depths would require including transverse spreading of the collimated beam. 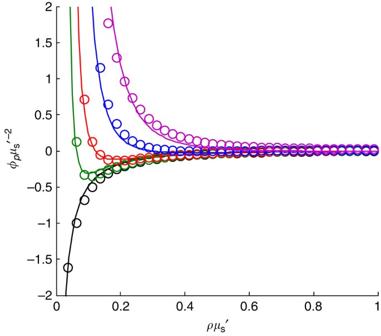Figure 4: Comparison of the PFC for internal fluence rate with the MC simulations. The PFC to the fluence rate within the medium (solid lines) is calculated for the H–G phase function withg=0.9. The MC data (circles) are obtained taking the difference in the fluence rate from a simulation with isotropic scattering (g=0) and a simulation withg=0.9. In all cases,0.001. The depth valuescorresponding to the colours black, green, red, blue and magenta are 0.01, 0.06, 0.1, 0.24 and 0.5, respectively. Figure 4: Comparison of the PFC for internal fluence rate with the MC simulations. The PFC to the fluence rate within the medium (solid lines) is calculated for the H–G phase function with g =0.9. The MC data (circles) are obtained taking the difference in the fluence rate from a simulation with isotropic scattering ( g =0) and a simulation with g =0.9. In all cases, 0.001. The depth values corresponding to the colours black, green, red, blue and magenta are 0.01, 0.06, 0.1, 0.24 and 0.5, respectively. 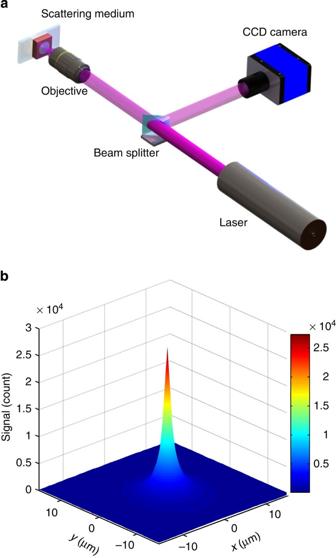Figure 5: Experimental schematic and spatially resolved reflectance. Schematic of the experimental setup. The expanded incident laser beam passes through a 20/80 beamsplitter and is delivered to the scattering sample through an objective. Light scattered from the sample is collected by the same objective and is reflected by a beamsplitter toward the imaging CCD. (b) Experimentally collected spatially resolved reflectance. Full size image Comparison with experimental measurements We also compared the reflectance calculated using PFC with experimental measurements performed using the setup shown in Figure 5a (see Methods for details). A high numerical aperture (NA) objective was used in this setup because equations (6) and (7) describe a 2 π collection solid angle, and the MC simulations show the illumination NA has virtually no effect on the shape of the reflectance near the POE ( Supplementary Fig. S3 ). The scattering medium consisted of a mixture of an aqueous glycerine solution and polystyrene microspheres with a diameter of 0.457 μm (Polysciences, Inc.). Using the Mie theory [34] and assuming a Gaussian size distribution of the microspheres with a s.d. of 0.011 μm, as listed by the manufacturer, we calculated the reduced scattering coefficient of the scattering sample to be =5.6 mm −1 and the anisotropy factor to be g =0.89. The absorption coefficient of the scattering sample is approximately μ a =0.001 mm −1 (see Methods for details). The reflectance signal measured from the polystyrene microsphere sample is presented in Figure 5b . We note that the measurements were performed tens of micrometres from the POE, where the signal strength has significant variation. This distance is comparable to cellular sizes in biological tissue. Thus, measurements of the reflectance from tissue on this scale could be sensitive to alterations in cell architecture associated with normal function or early, pre-cancerous changes. Figure 5: Experimental schematic and spatially resolved reflectance. Schematic of the experimental setup. The expanded incident laser beam passes through a 20/80 beamsplitter and is delivered to the scattering sample through an objective. Light scattered from the sample is collected by the same objective and is reflected by a beamsplitter toward the imaging CCD. ( b ) Experimentally collected spatially resolved reflectance. 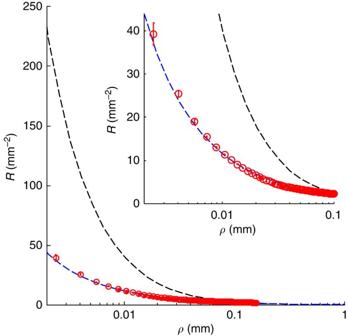Figure 6: Comparison with the experiment. Red circles—experiment, the bars on the experimental points show the range of measurements. Black dashed line—standard DA, blue dashed line—PFC diffusion theory. Inset: expanded view of the critical region near the POE to show the range of measurements more clearly. The PFC diffusion theory demonstrates excellent agreement with the experiment, whereas the DA deviates significantly near the POE. Full size image Figure 6 shows the experimental reflectance spectra and a comparison with the DA and PFC theories. Although the DA exhibits significant deviation from the experiment for distances smaller than 100 μm from the POE, PFC shows excellent agreement. Figure 6: Comparison with the experiment. Red circles—experiment, the bars on the experimental points show the range of measurements. Black dashed line—standard DA, blue dashed line—PFC diffusion theory. Inset: expanded view of the critical region near the POE to show the range of measurements more clearly. The PFC diffusion theory demonstrates excellent agreement with the experiment, whereas the DA deviates significantly near the POE. Full size image One of the major applications of this theory will be solving the inverse problem to obtain optical properties of unknown turbid samples, especially on a significantly smaller scale than it can be done presently. Fortunately, the same inversion techniques [35] , [36] that have been used with the standard DA to extract and μ a can be applied with the PFC, provided that adequate assumptions are made regarding the phase function. Aside from higher accuracy near the source, PFC also allows for the inversion of parameters of the phase function. For example, the anisotropy factor can be measured by assuming either Mie or the H–G scattering and using g as a free parameter in the fitting to experimental data. Moreover, the entire backscattering portion of the phase function can potentially be reconstructed. A requirement of the technique is the availability of an accurate isotropic solution ( g =0). Although this solution is available for diffuse reflectance, an accurate solution for the fluence rate near the POE is not commonly available. One approach for obtaining the fluence rate within the medium would be to use the MC simulation for isotropic scattering and combine it with PFC to obtain the fluence for arbitrary phase functions. This is the approach we used for obtaining the results in Figure 6 . Thus, the result of a single MC simulation can be used to obtain solutions for a large array of phase functions and anisotropy parameters. It is also likely that PFC could be used to describe angular dependences in a similar manner. In conclusion, the PFC diffusion theory for light transport in turbid media addresses the deficiencies of the standard diffusion theory near the POE by accounting for the specific form of the phase function. The technique accurately predicts the correct scattering behaviour for two frequently used but very different types of phase functions, the H–G and Mie theory phase functions ( Fig. 2a ). The PFC approach results in a substantial improvement over the predictions of the δ − P 1 approximation and the P 3 approximation ( Fig. 2b ), each of which seeks to improve the performance of the DA. PFC also demonstrates excellent agreement with experimental results ( Fig. 6 ). We anticipate that this work will be utilized extensively in characterizing photon scattering in turbid media such as human tissue and in a variety of other applications. Evaluation of the integral terms To evaluate the first integral term μ s ∫∫[ p ( s · s ′)− p DI ( s · s ′)] L d ( r , s ′) d s ′, we use the standard DA expression for L d ( r , s ) where φ d ( r ) is the fluence rate and is the current density [37] . By substituting in the integral, we get From here, we see directly that because of the unity normalization of both phase functions. Let us now simplify the integral term ∫∫ p ( s , s ′) ( s ′· j d ( r )) d s ′ and re-write it in a spherical coordinate system ( Fig. 7a ). The integral can be expressed as μ s | j d ( r )|∫∫ p (cos θ ) (sin θ j ·sin ϕ ·sin θ +cos θ ·cos θ j ) sin θ d θ d ϕ , where is the unit vector in the direction of vector j d ( r ), θ =cos −1 ( s · s ′), and . The part proportional to the sin θ j ·sin ϕ ·sin θ is zero as . The part proportional to cos θ ·cos θ j gives | j d ( r )|cos θ j ∫∫ p (cos θ ) cos θ sin θ d θ d ϕ . Here | j d ( r )|cos θ 0 = s · j d ( r ) and, by definition ∫∫ p (cos θ ) cos θ sin θ d θ d ϕ = g . Thus, we see that ∫∫ p ( s , s ′) ( s ′· j d ( r )) d s ′= g ( s · j d ( r )). 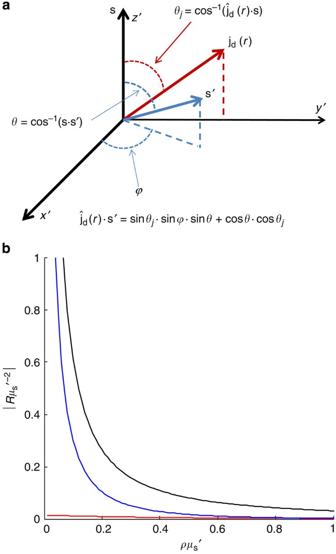Figure 7: Evaluation of the contribution of the neglected integral term. (a) Angles between vectorss,s′ andjd(r). The vectorsdefines thez′. The vectorssandjd(r) define the (y′,z′) plane. (b) Contributions of the neglected integral term, PFC term and diffuse reflectance term to the reflectance. Black line—radially dependent diffuse reflectanceRd(ρ), blue line—contribution of the PFC termRp(ρ), red line—contribution of the neglected integral term ΔRp(ρ). The contribution of the neglected integral term, ΔRp(ρ), is less than 4% ofRp(ρ) for. The contribution of ΔRp(ρ) is less than 7% ofRd(ρ) for. The calculations are performed for H–G phase function,g=0.9 and=0.01. By substituting this into the remaining portion of the integral we get Figure 7: Evaluation of the contribution of the neglected integral term. ( a ) Angles between vectors s , s ′ and j d ( r ). The vector s defines the z ′. The vectors s and j d ( r ) define the ( y ′, z ′) plane. ( b ) Contributions of the neglected integral term, PFC term and diffuse reflectance term to the reflectance. Black line—radially dependent diffuse reflectance R d ( ρ ), blue line—contribution of the PFC term R p ( ρ ), red line—contribution of the neglected integral term Δ R p ( ρ ). The contribution of the neglected integral term, Δ R p ( ρ ), is less than 4% of R p ( ρ ) for . The contribution of Δ R p ( ρ ) is less than 7% of R d ( ρ ) for . The calculations are performed for H–G phase function, g =0.9 and =0.01. Full size image as both phase functions p ( s · s ′) and p DI ( s · s ′) have the same anisotropy factor g . Thus, indeed μ s ∫∫[ p ( s · s ′)− p DI ( s · s ′)] L d ( r , s ′) d s ′=0. To evaluate the contribution of the second integral term μ s ∫∫[ p ( s · s ′)−(2π) −1 g · δ (1− s · s ′)] L p ( r , s ′) d s ′, we calculated the PFC to the radially-dependent reflectance including this integral. Then we subtracted R p ( ρ ) obtained by neglecting this integral to calculate Δ R p ( ρ ). We then plot Δ R p ( ρ ) and could see it is just several percent of R p ( ρ ) for small ( Fig. 7b ). We also included R d ( ρ ) to show that at greater both corrections are neglectable. Thus, neglecting μ s ∫∫[ p ( s · s ′)−(2π) −1 g · δ (1− s · s ′)] L p ( r , s ′) d s ′ is justified. Experimental setup A schematic of the experimental setup is shown in Figure 5a . The setup uses a confocal microscope (FluoView 1000, Olympus) with several modifications. The incident 458-nm laser beam is expanded to fill the back aperture of the objective and passes through a 20/80 beamsplitter (Chroma). The beam is delivered to the scattering sample through a planar apochromatic oil immersion objective (NA=1.32, ×63 magnification, Olympus). Light scattered from the sample is collected by the same objective and is reflected by a beamsplitter towards the imaging lens and the imaging CCD (DU-434-FI, Andor Technology). The spatial scale for imaging the scattering sample is derived by calibrating the CCD with a counting chamber (Millipore), with a single CCD pixel imaged to 0.327 μm on the sample. Scattering sample The sample is placed in an imaging chamber assembled from a glass slide, four adhesive silicone isolators (JTR20R-A2-1.0, Grace Bio-Labs Inc.), and a No. 1 cover glass. The resulting chamber had a 20-mm internal diameter and a 4-mm depth. We placed optical gel (LS-3238, Fibre Optic Centre) on the inside surface of the cover glass. After curing, the optical gel formed a layer of ∼ 0.1 mm thickness with a refractive index of 1.388. The same refractive index of 1.388 at the 458-nm wavelength is achieved in the scattering sample by mixing a 66% volume fraction of the polystyrene microspheres aqueous solution and a 34% volume fraction of glycerine [38] . By matching indices we minimize the effects of specular reflection and obtain a matched boundary condition at the interface. The absorption coefficient of the sample can be estimated as a weighted average of the absorption coefficients of the glycerine, water and polystyrene in the sample. The absorption coefficient of water [39] at the wavelength 458 nm is 2.7×10 −5 mm −1 . The absorption coefficient of glycerol [40] is ∼ 0.003 mm −1 and the absorption coefficient of polystyrene [41] is less than 1×10 −5 mm −1 . Thus, the absorption coefficient of the scattering sample is ∼ 0.001 mm −1 . How to cite this article: Vitkin, E. et al . Photon diffusion near the point-of-entry in anisotropically scattering turbid media. Nat. Commun. 2:587 doi: 10.1038/ncomms1599 (2011).